Prevalent mutator genotype identified in fungal pathogenCandida glabratapromotes multi-drug resistance The fungal pathogen Candida glabrata has emerged as a major health threat since it readily acquires resistance to multiple drug classes, including triazoles and/or echinocandins. Thus far, cellular mechanisms promoting the emergence of resistance to multiple drug classes have not been described in this organism. Here we demonstrate that a mutator phenotype caused by a mismatch repair defect is prevalent in C. glabrata clinical isolates. Strains carrying alterations in mismatch repair gene MSH2 exhibit a higher propensity to breakthrough antifungal treatment in vitro and in mouse models of colonization, and are recovered at a high rate (55% of all C. glabrata recovered) from patients. This genetic mechanism promotes the acquisition of resistance to multiple antifungals, at least partially explaining the elevated rates of triazole and multi-drug resistance associated with C. glabrata . We anticipate that identifying MSH2 defects in infecting strains may influence the management of patients on antifungal drug therapy. C andida species account for the most mucosal and invasive fungal infections worldwide [1] and are the fourth leading cause of nosocomial bloodstream infections in the United States [2] . Candida bloodstream infections cause estimated healthcare costs of $2–4 billion per year in the United States alone and are associated with a crude mortality rate of 40%, even with antifungal treatment [1] . The current arsenal of antifungal drugs is limited, with only two non-toxic antifungal classes to treat candidiasis: triazoles (for example, fluconazole and voriconazole) and echinocandins (for example, caspofungin and micafungin). Polyenes, such as amphotericin B formulations, represent a third class of antifungals, but polyene use is more restricted due to nephrotoxicity [3] . Although 50% of worldwide candidemia cases are caused by C. albicans , there has been a steady shift towards non-albicans species over the past 20 years [1] , [4] . In North America, C. glabrata now accounts for ∼ 25% of Candida infections [4] , [5] . Albeit this species lacks some important Candida virulence factors, including hyphal formation, between 20 and 30% of C. glabrata strains exhibit triazole resistance, and this number continues to rise [6] , [7] . C. glabrata has also developed resistance to the echinocandins, which were introduced into the market less than 15 years ago, at a faster rate than any other Candida species [6] . Depending on the study and geographical location, between 3 and 12% of C. glabrata isolates now demonstrate resistance to one or more echinocandin [6] , [8] . Alarmingly, multi-drug resistant (MDR) C. glabrata [6] , [8] , [9] , [10] , [11] , [12] , which exhibit resistance to two or more classes of antifungal drugs, are commonly encountered leaving virtually no options for treatment. Different antifungal drug classes have distinct targets and mechanisms of action and resistance [13] , and it is unclear why C. glabrata is capable of rapidly acquiring resistance to multiple drug classes. The acquisition of resistance frequently observed with C. glabrata has historically been ascribed to its haploid genome. We hypothesized that a defect in DNA repair may account for accelerated emergence of various genetic changes responsible for drug resistance. Normally, DNA repair is responsible for correcting errors made by DNA polymerase during DNA replication, as well as for repairing DNA damage caused by environmental factors, such as chemicals or radiation, or by endogenous factors, such as reactive oxygen radicals. Thus far, the role of DNA repair in fungal pathogens, especially in the emergence of antifungal resistance, has not been explored in depth. Here we focused on the role of two DNA repair pathways in C. glabrata —mismatch repair (MMR) and double-strand break repair (DSBR)—because defects in these pathways in bacteria [14] ( in vitro and in vivo ) and C. albicans [15] ( in vitro ) have been shown to lead to a hyper-mutable phenotype. More specifically, homozygous disruption of DSBR gene RAD50 and MMR genes MSH2 and PMS1 in C. albicans led to an elevated frequency of fluconazole-resistant colonies [15] ; therefore, we began our studies examining homologous genes in C. glabrata . We found that disruption of MSH2 in C. glabrata led to a hyper-mutable phenotype and significant increases in the emergence of antifungal resistant mutants. Nonsynonymous mutations discovered within MSH2 in over half (195 out of 357) of the clinical strains analyzed produced similar phenotypes. Our data suggest that defects in mismatch repair represent a key, underlying cellular mechanism that facilitates emergence of resistance to multiple antifungals in C. glabrata . MSH2 deletion leads to an increase in resistant mutants To determine the effects of DNA MMR and DSBR on C. glabrata antifungal resistance, we separately disrupted one MMR gene, MSH2 (CAGL0I07733g) and one DSBR gene, RAD50 (CAGL0J07788g). 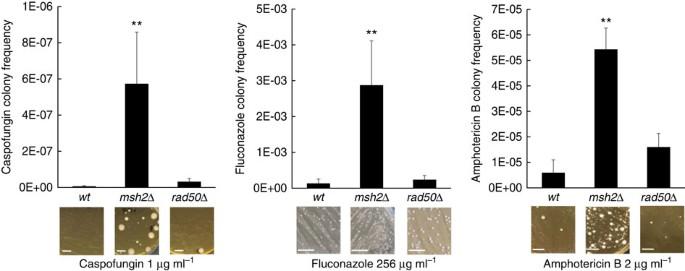Figure 1: Deletion ofMSH2inC. glabrataleads to significantly more resistant colonies upon selection on multiple antifungal drugs. Wild type,msh2Δandrad50Δstrains were selected on media containing caspofungin (an echinocandin), fluconazole (a triazole) and amphotericin B (a polyene) at concentrations from 16- to 32-fold greater than wild type MICs as described in Methods section. The plots show means of resistant colony frequencies from ≥3 independent experiments±s.d. SeeSupplementary Fig. 1for resistant frequencies to voriconazole (triazole) and micafungin (echinocandin). **P<0.01 (student’st-test; two-tailed). Representative images of selection plates are shown. Scale bars=1 cm. Echinocandin and fluconazole minimum inhibitory concentrations (MICs) were not significantly changed (<2-fold) in the disruptants when compared with the wild type parental strain ( Supplementary Table 1 ). However, subsequent antifungal selections revealed that the msh2Δ strains generated ∼ 82-, 18- and 9-fold more caspofungin-, fluconazole- and amphotericin B-resistant mutants, respectively, when compared with the wild type strain ( Fig. 1 ). The rad50Δ strain did not affect antifungal resistance frequencies as strongly (2 to 5-fold increases relative to wild type). The msh2Δ strain also exhibited increased resistance frequencies to micafungin and voriconazole ( Supplementary Fig. 1 ). Over 90% of echinocandin- (caspofungin and micafungin) selected colonies displayed high-level resistance (MICs>2 μg ml −1 ) and 100% of those resistant msh2Δ colonies (25/25) displayed a hotspot mutation in either Fks1 or Fks2 ( Table 1 ). Fks1/2 hotspot mutations represent the primary mechanism of echinocandin clinical resistance [16] . C. glabrata triazole resistance arises most commonly through overexpression of drug efflux pumps, which is achieved through gain-of-function mutation of the transcription factor Pdr1 (refs 17 , 18 ). As expected, pdr1 mutations were identified in 10 of 14 fluconazole-resistant wild type and msh2Δ mutants ( Table 1 ). Likewise, an erg6 mutation (Erg6-K157fs) was identified in one amphotericin B-resistant mutant from msh2Δ selections ( Table 1 ). Compared with triazoles and echinocandins, molecular mechanisms of polyene resistance are less well described in C. glabrata ; however mutations in specific ERG genes, including ERG6 have been associated with polyene reduced susceptibility [19] , [20] . These data show that defects in MMR facilitate the emergence of mechanistically diverse C. glabrata antifungal drug resistance in vitro . Figure 1: Deletion of MSH2 in C. glabrata leads to significantly more resistant colonies upon selection on multiple antifungal drugs. Wild type, msh2Δ and rad50Δ strains were selected on media containing caspofungin (an echinocandin), fluconazole (a triazole) and amphotericin B (a polyene) at concentrations from 16- to 32-fold greater than wild type MICs as described in Methods section. The plots show means of resistant colony frequencies from ≥3 independent experiments±s.d. See Supplementary Fig. 1 for resistant frequencies to voriconazole (triazole) and micafungin (echinocandin). ** P <0.01 (student’s t -test; two-tailed). Representative images of selection plates are shown. Scale bars=1 cm. Full size image Table 1 Mutation or disruption of MSH2 leads to increases in resistance-conferring mutations. Full size table msh2 mutations identified in diverse clinical isolates To investigate whether defects in MMR contribute to emergence of antifungal resistance in the clinic, we acquired 357 geographically diverse C. glabrata strains, including 66 from Duke Hospital (Durham, NC), 118 from the Centers for Disease Control (Atlanta, GA), 25 from MD Anderson Cancer Center (Houston, TX), 18 from Wayne State University Medical School (Detroit, MI), 40 from the University Hospital at Lausanne (Switzerland), 74 from Hamad Medical Corporation (Qatar) and 17 miscellaneous strains from the laboratory collection of one of the authors (D.S.P.). MSH2 was sequenced in all strains. Overall, 55% of these strains contained a nonsynonymous mutation within Msh2 when compared with the database strain, CBS138/ATCC2001 ( http://www.candidagenome.org/ ). We further assigned these strains into one of four categories: susceptible, fluconazole-resistant (fluconazole R ), echinocandin-resistant (echinocandin R ) or MDR (both fluconazole R and echinocandin R ). Resistant MICs were defined according to the standards recommended by the Clinical and Laboratory Standards Institute (CLSI) [21] , [22] . We do note that although a fluconazole MIC of 32 μg ml −1 is defined as susceptible dose dependent, we included these isolates in the fluconazole R group. Seventy-four out of the 81 fluconazole R -classified isolates sequenced (all groups except Hamad Medical Corporation) contained a Pdr1 mutation ( Supplementary Data 1 ). Single mutations of specific amino acids in Pdr1, including V329, N768, P927 and T1080, were identified in both clinical isolates and lab-generated mutants ( Table 1 and Supplementary Data 1 ). Echinocandin resistance was declared if an isolate demonstrated a resistant MIC to at least two of the three echinocandin drugs. Forty-five of the 47 echinocandin R -classified isolates (echinocandin R and MDR groups) contained an Fks1 or Fks2 hotspot mutation ( Supplementary Data 1 ). Out of the 357 clinical strains analyzed, 52% (117/225) of susceptible isolates demonstrated a nonsynonymous mutation within Msh2, while a mutation was discovered in 65% of fluconazole R isolates (54/83; P <0.05 versus susceptible, χ 2 =4.1879) and 62% of MDR isolates (21/34; ns versus susceptible, χ 2 =1.1314) ( Fig. 2a,b ). We did find individual center differences. For example, strains from Duke Hospital exhibited similar levels of msh2 mutations in susceptible (53%), fluconazole R (46%) and MDR isolates (50%) ( Fig. 2b ), whereas isolates obtained from other centers (MD Anderson Cancer Center and University Hospital at Lausanne) demonstrated a pattern consisting of lower levels of mutations in susceptible isolates (29 and 52%) compared with fluconazole R isolates (100 and 73%, both respectively) ( Fig. 2b ). The only center that provided non-blood stream isolates, Wayne State University Medical School, demonstrated high levels of msh2 mutations in both susceptible and fluconazole R isolates (78% each). These vaginal isolates were obtained from patients with recurrent vaginitis. We found a low percentage of msh2 mutations in echinocandin R isolates, although fewer of these isolates were obtained ( Fig. 2b ). Overall, these data revealed that polymorphisms in the MSH2 gene are present in an unexpectedly high percentage of clinical C. glabrata isolates, particularly fluconazole R strains. 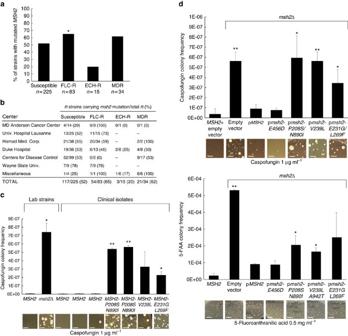Figure 2: Msh2 alterations identified in diverse clinical isolates cause a mutator phenotype and increased emergence of antifungal resistance. (a) The 357 clinical isolates obtained were classified according to their susceptibilities to fluconazole (FLC) and the echinocandins (ECH), and the percentage of isolates within each group demonstrating a nonsynonymousmsh2mutation were determined.Pvalue was determined throughχ2analysis (compared with susceptible group). (b) All isolates were categorized by institution. Isolates demonstrating anmsh2mutation/total isolates are shown for each susceptibility group. SeeSupplementary Data 1for a list of all individual isolates analyzed. (c) Echinocandin- (caspofungin) resistant colony frequencies of various clinical isolates were measured. (d) Wild type ormsh2Δcells expressing an empty orMSH2-containing plasmid were selected on caspofungin and 5-fluoroanthranilic acid. SeeSupplementary Table 4for strains. Frequency data inc,dare mean±s.d. from three independent experiments; representative images are shown. *P<0.05, **P<0.01 (student’st-test; two-tailed). Scale bars=1 cm. Figure 2: Msh2 alterations identified in diverse clinical isolates cause a mutator phenotype and increased emergence of antifungal resistance. ( a ) The 357 clinical isolates obtained were classified according to their susceptibilities to fluconazole (FLC) and the echinocandins (ECH), and the percentage of isolates within each group demonstrating a nonsynonymous msh2 mutation were determined. P value was determined through χ 2 analysis (compared with susceptible group). ( b ) All isolates were categorized by institution. Isolates demonstrating an msh2 mutation/total isolates are shown for each susceptibility group. See Supplementary Data 1 for a list of all individual isolates analyzed. ( c ) Echinocandin- (caspofungin) resistant colony frequencies of various clinical isolates were measured. ( d ) Wild type or msh2Δ cells expressing an empty or MSH2 -containing plasmid were selected on caspofungin and 5-fluoroanthranilic acid. See Supplementary Table 4 for strains. 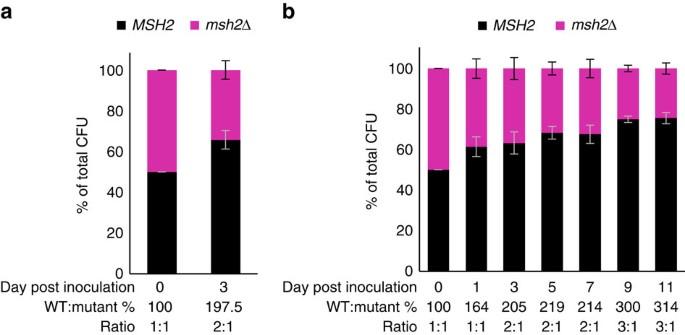Figure 4: Wild type cells partially outcompetemsh2Δin mixed inoculation mouse models. DNA was isolated from kidney tissue of systemically infected, immunosuppressed mice (a) and from fecal samples of GI-colonized, immune competent mice (b) and then subjected to SYBR green quantitative PCR with strain specific primers. Wild type (WT) to mutant ratios were calculated from qPCR DNA copy numbers. Means±s.d. are calculated. Frequency data in c , d are mean±s.d. from three independent experiments; representative images are shown. * P <0.05, ** P <0.01 (student’s t -test; two-tailed). Scale bars=1 cm. Full size image To better understand the timeline of appearance of these msh2 polymorphisms, we obtained and analyzed paired sets of isolates from the participating centers. Each pair (or triplet) of isolates was isolated from the same patient. Out of these 30 sets of isolates, 20 contained an msh2 mutation in at least one isolate ( Table 2 ). In all but three sets of isolates that contained an alteration, the identified mutation was present in all isolates from that patient, independent of the susceptibility, suggesting that the msh2 mutation predated the emergence of fluconazole and/or echinocandin resistance in these patients. Interestingly, in the remaining three sets (all from a single center), we identified differences in Msh2 within isolates taken from the same patient ( Table 2 ). In each case, an msh2 mutation or additional mutation(s) was only identified within the second, fluconazole R isolate ( Table 2 ). Table 2 Paired patient isolates containing msh2 mutations. Full size table Notably, 96% of msh2 mutations in the analyzed clinical isolates contained the following amino acid changes: P208S/N890I, E231G/L269F, V239L/A942T or V239L (see Supplementary Data 1 ). These amino acids (P208, E231, V239 and L269) map to the protein’s connector region, which is essential for interaction between the MutS (Msh2-Msh3/6) and MutL (Pms1-Mlh1) complexes and therefore, MMR activity [23] . Indeed, upon caspofungin selection in vitro , echinocandin susceptible clinical isolates containing these msh2 mutations produced significantly higher frequencies of echinocandin R colonies and fks mutants than isolates carrying wild type MSH2 ( Fig. 2c and Table 1 ). To directly analyze the functionality of the most commonly identified msh2 mutations, alleles were amplified from clinical isolates, expressed on a yeast centromere plasmid under the control of their native promoter, and transformed into a laboratory strain carrying a deletion of MSH2 . Forward mutation frequencies were analyzed by measuring frequencies of colonies resistant to the echinocandin caspofungin (largely due to mutations in FKS1 or FKS2 ) or to 5-fluoroanthranilic acid (5-FAA; largely due to mutations in TRP3 or TRP5 ) [24] . As expected, we found that msh2Δ exhibited a hyper-mutable phenotype (average caspofungin R colony frequency=5.63 × 10 −7 , average 5-FAA R colony frequency=5.32 × 10 −4 ; Fig. 2d ). While MSH2 derived from a wild type strain or from a clinical isolate containing one conservative mutation (E456D) complemented the msh2Δ mutant phenotype, expression of either msh2-P208S/N890I , msh2-V239L or msh2-E231G/L269F did not complement msh2Δ : the plasmid-borne msh2 alleles produced the high frequencies of echinocandin R and 5-FAA R colonies characteristic of the msh2Δ mutant ( Fig. 2d ). The resulting echinocandin R colonies contained Fks mutations, specifically fks1-S629P , fks2-S663P , fks2-S663Y and fks2-S663F ( Table 1 ), all of which have been previously shown to lead to echinocandin treatment failure [25] , [26] , [27] . Also, ∼ 25% of the 5-FAA R colonies contained trp3 nonsynonymous mutations ( Supplementary Table 2 ). Together, these data suggest that clinical strains of C. glabrata carry mutations in MSH2 , which result in MMR defects and promote the emergence of antifungal resistance. Colonization with msh2Δ leads to increased resistance in vivo To determine if altered MMR activity can promote the development of C. glabrata antifungal resistance in vivo , we utilized a mouse model of C. glabrata gastrointestinal (GI) colonization ( Fig. 3a ). This model recapitulates pathogenesis of human disease through overgrowth of yeast in the primary reservoir (GI). First, bacterial flora were eradicated from the GI tract with a daily piperacillin-tazobactam (PTZ) regimen [28] ( Fig. 3a ). Mice were then orally inoculated with either a wild type or msh2Δ strain followed by daily, sub-inhibitory echinocandin (caspofungin; 0.5 mg kg −1 i.p.) or vehicle (saline i.p.) administration for 21 days. Mice were effectively colonized (range: 5 × 10 7 to 1 × 10 8 CFU per gram of stool) with both the wild type and msh2Δ strains from days 1 to 27 post-inoculation ( Fig. 3a ). Of note, no significant growth difference between these strains in vitro was observed ( Supplementary Fig. 2 ). Caspofungin resistant colony frequencies from each mouse were tracked at one time point prior to and four time points following treatment initiation over a period of 18 days. While we observed no increases in resistant yeast recovered from eight caspofungin-treated mice that were colonized with the wild type strain, five of eight caspofungin-treated mice that were colonized with the msh2Δ strain demonstrated an increase in resistant colonies 6 to 12 days following treatment initiation, representative of an expanding fks mutant population ( Fig. 3b ). DNA sequencing revealed that echinocandin resistance was due to fks1 mutations in yeast recovered from those mice ( Fig. 3c ). 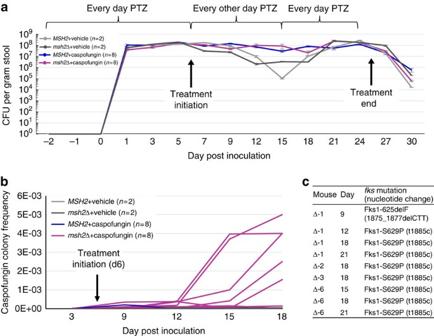This suggests that loss of MMR in C. glabrata can lead to an increased frequency of resistance-conferring mutations in vivo . Figure 3: Colonization withmsh2Δleads to increased echinocandin-resistancein vivo. (a) GI colonization of CF-1 mice represented through fecalC. glabrataburdens. Daily administration (i.p.) of caspofungin (CSF; 0.5 mg ml−1) or saline occurred from days 6 to 26 post-inoculation. (CSF-treated groups:n=8 wild type inoculated mice, 8msh2Δinoculated mice; Saline-treated groups:n=2 wild type, 2msh2Δ). Means±s.d. are calculated. (b) Fecal samples from each mouse at days 3, 9, 12, 15 and 18 (−3, 3, 6, 9 and 12 days post-treatment initiation, respectively) were selected on caspofungin (2 μg ml−1) containing YPD media (see Methods section for additional details). Five of eight CSF-treated mice that were inoculated withmsh2Δdemonstrated increase in resistant colony frequencies between days 12 and 18. (c)fks1mutants identified within fecal isolates. Colonies on antifungal-free plates (produced in parta) were replica plated onto caspofungin-containing media. Hotspot regions ofFKS1andFKS2(echinocandin drug targets) were amplified and sequenced in resistant colonies. Figure 3: Colonization with msh2Δ leads to increased echinocandin-resistance in vivo . ( a ) GI colonization of CF-1 mice represented through fecal C. glabrata burdens. Daily administration (i.p.) of caspofungin (CSF; 0.5 mg ml −1 ) or saline occurred from days 6 to 26 post-inoculation. (CSF-treated groups: n =8 wild type inoculated mice, 8 msh2Δ inoculated mice; Saline-treated groups: n =2 wild type, 2 msh2Δ ). Means±s.d. are calculated. ( b ) Fecal samples from each mouse at days 3, 9, 12, 15 and 18 (−3, 3, 6, 9 and 12 days post-treatment initiation, respectively) were selected on caspofungin (2 μg ml −1 ) containing YPD media (see Methods section for additional details). Five of eight CSF-treated mice that were inoculated with msh2Δ demonstrated increase in resistant colony frequencies between days 12 and 18. ( c ) fks1 mutants identified within fecal isolates. Colonies on antifungal-free plates (produced in part a ) were replica plated onto caspofungin-containing media. Hotspot regions of FKS1 and FKS2 (echinocandin drug targets) were amplified and sequenced in resistant colonies. Full size image Fitness of msh2Δ assayed in mixed inoculation mouse models In patients, strains containing defects in MMR may coexist with strains with wild type MMR function. Therefore, we performed fitness assays using both the aforementioned GI colonization model, as well as a systemic infection mouse model to assess the fitness of a MMR-deficient strain in vivo (see Methods section for details). Mice were inoculated with either wild type, msh2Δ , or an equal CFU mix of both strains. In the systemic model, kidneys were harvested at day 3 post-infection and subject to CFU plating and qPCR analysis following DNA isolation. Specific primers were designed for both wild type and msh2Δ strains ( Supplementary Table 3 ). SYBR green real-time PCR was used to quantify DNA copy number and calculate strain ratios. Similarly, fecal samples collected from colonized mice at day 1, 3, 5, 7, 9 and 11 post-inoculation were assessed for mixed population ratio. In the systemic infection model, the average wild type to mutant ratio found in kidneys isolated from mice infected with both strains was 2:1 ( Fig. 4a ), indicating a modest fitness defect of the msh2Δ strain. Similarly, we found an increasing wild type to mutant ratio in fecal samples over the course of the colonization model ( Fig. 4b ). Importantly, both models demonstrated similar levels of colonization and infection when inoculated with either wild type or msh2Δ alone ( Supplementary Fig. 3 ). Figure 4: Wild type cells partially outcompete msh2Δ in mixed inoculation mouse models. DNA was isolated from kidney tissue of systemically infected, immunosuppressed mice ( a ) and from fecal samples of GI-colonized, immune competent mice ( b ) and then subjected to SYBR green quantitative PCR with strain specific primers. Wild type (WT) to mutant ratios were calculated from qPCR DNA copy numbers. Means±s.d. are calculated. Full size image While antifungal drug resistance is nearly always due to fungal genome alterations ranging from point mutations to gain or loss of whole chromosomes [13] , the identity of specific DNA repair pathways that impinge on the emergence of C. glabrata resistance has remained unknown. Here, we have shown that an unexpectedly high percentage (55%) of clinical C. glabrata isolates carry loss-of-function mutations in the MMR gene MSH2 , which produced a mutator phenotype resulting in accelerated emergence of antifungal drug resistance both in vitro and in vivo . Interestingly, these mutations were more frequent among fluconazole R and MDR C. glabrata isolates ( Fig. 2a ), suggesting that their appearance may be associated with fluconazole exposure. While msh2 mutations were also found in nearly half of all drug susceptible isolates, we must emphasize that many patients were severely ill and had most likely been exposed to multiple drugs, including antibiotics, steroids, antineoplastics and/or antifungals, which may have also influenced the frequency of msh2 mutations. Differences in patient populations and antifungal administration practices are likely responsible for the significant discrepancies observed in the frequencies of msh2 mutations in susceptible and resistant isolates across different institutions ( Fig. 2a,b ). The lower percentage of msh2 mutations identified in echinocandin R clinical isolates may be due to a small number of such strains available for analysis. Alternatively, we cannot exclude a negative genetic interaction between defects in MMR and fks1/2 mutations, resulting in a fitness defect. Fks1-S629P was the primary mutation identified from the stool of echinocandin-treated mice colonized with msh2Δ ( Fig. 3c ), and the most frequent fks1 mutation among C. glabrata MDR clinical isolates with MMR defects ( Supplementary Data 1 ). Whether this mutation is associated with MDR and/or influences C. glabrata fitness remains to be investigated. The equivalent C. glabrata mutation in Fks2 (S663P) was recently shown to limit the macrophage inflammatory response upon caspofungin exposure, suggesting certain fks mutations have a higher propensity for immune evasion [29] , similar to pdr1 mutations [30] . The observation that only a limited spectrum of msh2 mutations were recovered from a large and diverse patient population may indicate that these mutations did not arise de novo in different patients, but that they pre-existed and were enriched for during drug treatment or pathogenesis (that is conversion from colonizer to infectious strain), perhaps by conferring a selective advantage under those conditions. This hypothesis is consistent with reports indicating that a mutator phenotype may be advantageous for fungal microevolution and survival within the host [31] . Also, the scenario where C. glabrata strains defective in MMR coexist with wild type strains in the host is consistent with our observation that the msh2Δ strain had only a mild fitness disadvantage in vivo when present together with the wild type strain ( Fig. 4 ). This fitness defect may result from the accumulation of mutations in essential genes; however, in single challenge studies, the msh2Δ strain exhibited comparable or slightly higher levels of colonization and infection relative to wild type ( Supplementary Fig. 3 ). Indeed, given that over half of our patient samples, including nearly half of all susceptible isolates, contain msh2 loss-of-function mutations, we suspect msh2 mutant colonizing strains have adapted well to their host, possibly though acquisition of gain-of-fitness mutations (for example, pdr1 mutation [32] ). Previously described fungal mechanisms of genetic instability that generate genetic diversity under stress have primarily involved gross chromosomal rearrangements and/or aneuploidy [33] . In contrast, our study presents the first example of a clinical, fungal population carrying a mutator phenotype due to genetic defects in a specific DNA repair pathway, namely MMR. It is possible that this mechanism of genetic instability is specific to C. glabrata because, unlike the other prevalent Candida species ( C. albicans , C. parapsilosis , C. tropicalis and C. krusei ), C. glabrata is a haploid organism where a single DNA repair mutation is sufficient to cause an associated mutator phenotype and subsequent emergence of resistance-conferring mutation(s). We suggest that the elevated levels of both triazole and multi-drug resistance associated with C. glabrata are at least partially due to the presence of msh2 mutations. Based on our results, by the time a patient requires administration of an antifungal, there is a substantial chance that the infecting strain contains an msh2 mutation. Therefore, we propose that C. glabrata MSH2 may be used as a biomarker prior to and throughout the course of therapy to determine the propensity of any given C. glabrata isolate to generate drug-resistant mutants and break through antifungal treatment. Thus, our study may have implications for antifungal prophylaxis, recurrent and long-term therapies, and antifungal stewardship protocols. Ethics statement Mice were housed in Public Health Research Institute’s Animal Biosafety Level-2 Research Animal Facility (ICPH RAF), a center of the New Jersey Medical School, Rutgers University (NJMS-Rutgers). Our animal facility follows the Public Health Service and National Institute of Health Policy of Humane Care and Use of Laboratory Animals. All experimental protocols were approved by the Rutgers Institutional Animal Care and Use Committee (IACUC). Strains and media A total of 357 C. glabrata clinical strains were obtained from patients with C. glabrata bloodstream or vaginal infections, including 66 from Duke Hospital (Durham, NC), 118 from the Centers for Disease Control (Atlanta, GA, USA), 25 from MD Anderson Cancer Center (Houston, TX, USA), 18 from Wayne State University Medical School (Detroit, MI, USA), 40 from the University Hospital at Lausanne (Switzerland), 74 from Hamad Medical Corporation (Qatar) and 17 additional miscellaneous strains from the laboratory collection of one of the authors (D.S.P.). Miscellaneous strains were obtained from the American Type Culture Collection (ATCC), Seongmin Lee (University of Texas), Hector Bonilla (Summa Health Systems), Barbara Alexander/Rachel Addison (Duke University), Marion Tuohy (Cleveland Clinic) and Soo-Hyun Kim (Chonnam National University Medical School) ( Supplementary Data 1 ). Entire or partial MIC and/or Fks mutational data from Duke University [6] , CDC [11] and S.H. Kim [12] (‘miscellaneous’ group) isolates have been previously published. The University Hospital at Lausanne isolates were all collected between the years of 1993 and 1996, predating echinocandin clinical use. Hotspots of the FKS1 and FKS2 genes were sequenced in echinocandin-resistant isolates. PDR1 was sequenced in fluconazole-resistant and select fluconazole-sensitive isolates from each collection except the Hamad Medical Corporation isolates. MSH2 was sequenced in all isolates. See Supplementary Table 3 for primers. Plasmid pGRB2.0 was obtained from Brendan Cormack (John’s Hopkins University School of Medicine) [34] . Yeast strains were maintained in YPD (1% yeast extract, 2% peptone and 2% dextrose) or synthetically-defined media lacking uracil (SD-ura) or tryptophan (SD-trp) (dropout base plus complete supplement mixture minus uracil or tryptophan). Plasmid-bearing DH5α E. coli strain was maintained in 40 μg ml −1 ampicillin-supplemented Luria-Bertani (LB) media. Plasmid-bearing C. glabrata strains ( Supplementary Table 4 ) were maintained in SD-ura media. Gene disruption and cloning C. glabrata ATCC 200989 (2001 HTU) or 2001 HTL (ref. 35 ) (gift from Karl Kuchler, University of Vienna) was transformed with a PCR-amplified TRP1 deletion cassette (see Supplementary Table 3 for primers). The deletion primers contain flanking regions that are homologous to the immediate up- and down-stream regions of each target gene’s coding region. Transformed cells were selected on synthetically-defined media lacking tryptophan, and colonies were PCR-screened and sequenced to confirm disruption. For plasmid-based expression of MSH2 , a gap-repair approach was used [36] . Briefly, coding regions plus promoter regions were PCR-amplified from laboratory or clinical isolates with primers ( Supplementary Table 3 ) containing flanking regions homologous to regions upstream and downstream of the SmaI restriction site in pGRB2.0. Strain 2001 HTU or msh2Δ were transformed with this PCR product, along with SmaI linearized pGRB2.0, and selected on SD-ura media. The resulting strains are listed in Supplementary Table 4 . Drug susceptibility assays Fluconazole and echinocandin minimum inhibitory concentrations (MICs) were determined by broth microdilution following CLSI standards as described [21] , [22] , except for the Qatar isolates, which were analyzed via Etest methodology according to the manufacturer’s instructions (Liofilchem, Italy). Fluconazole (LKT Laboratories, Saint Paul, MN), caspofungin (Merck, Rahway, NJ) and micafungin (Astellas, Deerfield, IL) were dissolved and diluted according to CLSI standards [21] . Fluconazole resistance was declared if an isolate demonstrated a CLSI-defined susceptible dose-dependent (32 μg ml −1 ) or resistant (≥64 μg ml −1 ) MIC, while echinocandin resistance was declared if an isolate demonstrated CLSI-defined resistance to at least two of the three echinocandins (≥0.5 μg ml −1 for caspofungin and anidulafungin, ≥0.25 μg ml −1 for micafungin). Drug selections and mutant analysis Strains were grown overnight in appropriate media (YPD or SD-ura) at 37 °C. We aimed to plate ∼ 1 × 10 8 CFU onto echinocandin-containing drug plates and between 1 × 10 5 and 1 × 10 6 CFU onto fluconazole, voriconazole (Pfizer), amphotericin B (Sigma-Aldrich, Milwaukee, WI) and 5-fluoroanthranillic acid (5-FAA, Sigma-Aldrich) plates. Drug concentrations of mutant selection plates were 16- to 32-fold greater than the wild type strain MICs. 5-FAA media was prepared as previously described [24] . A minimum of three biological replicate selections per strain were performed. Dilutions were plated onto drug-free media to determine exact CFU counts. Frequencies were calculated as number of colonies on the drug plate divided by the total CFU plated. Frequency averages were calculated from at least three independent selections from the concentration(s) indicated in Table 1 . Colonies were spotted onto plates containing two-fold higher drug concentrations and then appropriate target genes, for example, FKS1 hotspot 1, FKS2 hotspot 1, PDR1 , ERG6 and TRP5 , were PCR-amplified and sequenced in resistant colonies (see Supplementary Table 3 for primers). Colonization mouse model Six-week-old female CF-1 immunocompetent mice (Charles River Laboratories) were treated (s.c.) from day -2 to day 6 with 320 mg kg −1 PTZ(8:1) to clear native intestinal bacterial flora [28] . PTZ was then injected every other day (days 8, 10, 12, 14, 16) and returned to daily injections near the end of the experiment (days 17–25). On day 0, mice were inoculated via oral gavage with ∼ 1.5 × 10 8 CFU of C. glabrata 2001 HTL wild type or isogenic strain mshΔ ( Supplementary Table 4 ) in 100 μl of saline. Strain 2001 HTL was utilized instead of 2001 HTU (ATCC 200989) because the histidine, leucine and tryptophan auxotrophies do not significantly affect the fitness or virulence of C. glabrata [35] . Fresh fecal samples were collected throughout the experiment to assess fungal GI tract colonization. Fungal burden was determined by plating proper dilutions of fecal samples onto drug-free YPD plates and recorded as C. glabrata CFU per gram of stool. Daily administration of caspofungin (0.5 mg kg −1 ) or saline (100 ul i.p.) was initiated on day 6 post inoculation, when stabilized colonization was observed, and continued through day 26. Colonies on burden plates were replica-plated onto caspofungin (2 μg ml −1 ) plates and FKS1 and FKS2 hotspots were PCR-amplified and sequenced in those demonstrating resistance. Caspofungin-resistant colony frequencies were determined through selection of fecal samples on YPD plates supplemented with caspofungin (2 μg ml −1 ), PTZ (16 μg ml −1 ) and chloramphenicol (20 μg ml −1 ). The increased caspofungin resistant colony frequencies observed with the animal fecal selections are approximately a 3.7 log increase (5000 × ) from the caspofungin selection of the untreated msh2Δ strain (compare Fig. 1 with Fig. 3a ), allowing us to conclude that the expanded fks mutant populations within these mice account for that frequency difference. Nonetheless, replica-plating from drug-free plates was used to uncover fks mutants to ensure the mutant arose in the animal as opposed to on the plate. Fitness assays For the colonization fitness study, mice were colonized as above, but with an equal mix of C. glabrata 2001 HTL wild type and isogenic strain mshΔ totaling 1.5 × 10 8 CFU in 100 μl of saline. Control inoculum groups were colonized with 1.5 × 10 8 CFU of a single strain. PTZ treatment was administered daily from day -2 to day 11. Fecal samples were collected on days 0, 1, 3, 5, 7, 9 and 11. Plating of fecal material and CFU counts were performed as stated above. For DNA extraction, approximately half of the homogenized fecal pellet was subjected to a 2 h incubation with proteinase K (50 μg ml −1 ; Ambion) followed by purification with QIAamp DNA Mini Kit (Qiagen). DNA was isolated from the pellets of each mouse at each time point. DNA was then subjected to SYBR green quantitative PCR (qPCR) using strain-specific primers ( Supplementary Table 3 ) to determine copy number of each strain within the samples. SYBR green qPCR was performed on a Mx3005P real-time instrument (Agilent) using Rotor-Gene SYBR Green PCR kit (Qiagen). The thermal cycling conditions consisted of an initial activation step at 95 °C for 5 min and 35 cycles at 95 °C for 10 s, and 60 °C for 20 s, followed by a dissociation step at 95 °C for 1 min, ramping temperature from 55 to 95 °C at the rate of 0.2 °C s −1 . Specificity of the primers was confirmed by observing a single peak in the dissociation curve. The detection limit and amplification efficiency of both assays were evaluated by testing 10-fold diluted DNA series (10 ng ∼ 100 fg per reaction) for wild type, msh2Δ , 10:1 mix of wild type and msh2Δ , 1:1 mix of wild type and msh2Δ , and 1:10 mix of wild type and msh2Δ . The 1:1 mix of wild type and msh2Δ were also used as external standards for strain quantification in each animal sample testing run. For the systemic infection study, neutropenia was induced in 8-week-old BALB/c mice (Charles River Laboratories) through administration of 150 mg kg −1 cyclophosphamide i.p. on day -4 and 100 mg kg −1 on days -1 and day 2 post infection. Mice were challenged (i.v.) with an equal mix of C. glabrata 2001 HTL wild type and msh2Δ totaling 4.0 × 10 7 CFU in 100 μl of saline. Control groups were infected with 4.0 × 10 7 CFU of a single strain. On day 3 post infection, mice were euthanized and kidneys harvested. Half of each kidney was homogenized and dilutions plated for total CFU counts and the remaining halves were subjected to DNA isolation as stated above, except with an overnight proteinase K digestion. DNA was subjected to the same qPCR analysis as the fecal DNAs. Statistics All data analyses were performed using GraphPad Prism, version 5.0, software for Windows (GraphPad Software, San Diego, CA). χ 2 analysis was used to determine differences in msh2 mutational status between susceptibility groups. Differences of resistant frequency between strains were evaluated by Student’s t -test. A P value of <0.05 (two-tailed) is considered statistically significant. How to cite this article: Healey, K. R. et al . Prevalent mutator genotype identified in fungal pathogen Candida glabrata promotes multi-drug resistance. Nat. Commun. 7:11128 doi: 10.1038/ncomms11128 (2016).